Accessing topological superconductivity via a combined STM and renormalization group analysis The search for topological superconductors has recently become a key issue in condensed matter physics, because of their possible relevance to provide a platform for Majorana bound states, non-Abelian statistics, and quantum computing. Here we propose a new scheme which links as directly as possible the experimental search to a material-based microscopic theory for topological superconductivity. For this, the analysis of scanning tunnelling microscopy, which typically uses a phenomenological ansatz for the superconductor gap functions, is elevated to a theory, where a multi-orbital functional renormalization group analysis allows for an unbiased microscopic determination of the material-dependent pairing potentials. The combined approach is highlighted for paradigmatic hexagonal systems, such as doped graphene and water-intercalated sodium cobaltates, where lattice symmetry and electronic correlations yield a propensity for a chiral singlet topological superconductor. We demonstrate that our microscopic material-oriented procedure is necessary to uniquely resolve a topological superconductor state. The search for topological states of matter has recently generated a flurry of broad activity in the field of superconductivity (for several paradigmatic directions, see, refs 1 , 2 , 3 , 4 , 5 , 6 , 7 , 8 , 9 , 10 , 11 ). A topological superconductor (SC) is an unprecedented state of quantum matter, which possesses a full pairing gap in the bulk but gapless exotic surface states as well as possibly non-trivial vortex bound states [2] , [6] , [12] . A chiral SC [1] , [2] , [13] with broken time-reversal symmetry (TRS) may be considered the superconducting analogue of the quantum Hall phase (as characterized by a non-trivial Chern number of its Bogoliubov bands [14] ), whereas a topological SC conserving TRS [7] is closely related to the quantum spin Hall phase (along with its non-trivial invariant [15] ). Recently, chiral SCs have enjoyed significant attention, exhibiting a variety of exotic phenomena based on their non-trivial topology [1] , such as hosting Majorana vortex bound states [2] , [12] and gapless chiral edge modes, that carry quantized thermal or spin currents (see for example ref. 16 ). The Majorana bound states can be interpreted as elusive fermionic particles equivalent to their own antiparticles, and have potential applications in fault-tolerant topological quantum computation [17] . In view of these striking properties, it would be desirable to develop guidelines to identify materials with the potential to host chiral topological SC states. As it turns out, the interplay of the lattice symmetry, the shape and the size of the Fermi surface (fermiology), the multi-orbital character and the electron–electron interactions are decisive for an unconventional chiral pairing mechanism. Material-specific research into this direction first concentrated on the perovskite Sr 2 RuO 4 , where experimental evidence points to a chiral odd-parity p-wave SC state [18] , as a possible analogue of superfluid 3 He (ref. 19 ). However, the topologically protected Majorana edge modes, which should appear in the chiral p-wave SC when a half-quantum vortex is injected [12] , [20] , have—so far—not uniquely been identified, despite strong experimental efforts [21] . It suggests that the odd-parity pairing, along with its non-trivial spin dependence, induces challenges which in terms of complexity even overshadow the original task to identify a material with topological chiral SC. Therefore, the even-parity topological chiral SC states, like d+id topological SC states, are more promising. Although the edge states in d+id chiral SC are fermionic (with the Chern number for the Bogoliubov bands C =±2 (refs 22 , 23 , 24 )), one can engineer a d+id SC state using spin–orbit interactions and weak Zeeman fields to generate a Majorana edge state [25] , [26] , [27] . On a square lattice, where most unconventional superconductors are found, the difficulty in realizing such a d+id singlet state is that the generic fermiology and interactions, which can yield a d-wave state, favour over d xy pairing. This changes for hexagonal lattices, where the lattice symmetry protects the degeneracy of the -wave and the d xy -wave SC at the instability level. This then yields a chiral singlet —superconducting state below the critical temperature, T C , to maximize the condensation energy [27] , [28] . In contrast to p+ip odd-parity pairing, the singlet character of the unconventional pairing should make its emergence more generic, as it stems from electron-mediated pairing where large wave vector particle-hole fluctuations tend to drive singlet superconductivity. This has been recently addressed in several theoretical scenarios of a d+id state such as for doped graphene [29] , [30] , [31] , [32] , [33] , [34] , [35] (for a recent review see ref. 27 ), water-intercalated sodium cobaltates [36] , and the pnictide SC SrPtAs (ref. 37 ). Recent experiments [38] show that highly doped graphene close to the van Hove singularity (vHS) can be prepared. Still, superconductivity in graphene has not yet been experimentally confirmed. From this perspective, water-intercalated sodium cobaltates and the pnictide SrPtAs may be more promising because, in both of these compounds, superconductivity has been already discovered [39] , [40] . Furthermore, some indications of unconventional SC were observed in Knight shift data on cobaltates [41] , as well as in muon-spin rotation/relaxation measurements and nuclear quadrupole experiments on SrPtAs (refs 42 , 43 ). While no unambiguous experimental confirmation of chiral d-wave SC for these materials exists so far, further experimental attention is certainly warranted and could lead to the first unambiguous identification of chiral topological SC. A characteristic challenge in the search for unconventional chiral SC is the pronounced competition between different orders, such as spin-density wave (SDW) and different SC orders, in particular the TRS-broken d+id SC state and an f-wave state with TRS [28] , [44] on the hexagonal lattice. This clearly calls for methods, that are capable of distinguishing the competing channels at the instability level, this means at low energies of the order of the SC gap features. This is the main strength of the functional renormalization group (fRG) method (for reviews see refs 28 , 45 ), which allows for a systematic connection via renormalization between a high-energy bare Hamiltonian and a low-energy effective theory, where the SC channels can be resolved. Knowing the precise functional form of the pairing function from the fRG calculations is of fundamental importance to make contact with experimental signatures. Here we demonstrate, that a combination of the microscopic theory, which is the fRG method, with the theory of scanning tunnelling spectroscopy (STM) makes this connection between theory and experiment possible. Although the main task of our work is to elevate spectroscopic signatures to provide evidence in favour of a possible singlet chiral topological SC state, for the role-model systems graphene and cobaltates, our approach can be straightforwardly extended to other classes of topological SC and should pave the road to find Majorana fermions in these systems. The conventional STM theory has been successful in a variety of situations, where it has been viewed as a phenomenology, assuming a certain ansatz for an order parameter [46] , [47] , [48] . Here we show, that our microscopic material-oriented procedure is necessary in the case of competing anisotropic SC channels such as d+id and f-wave: the phenomenological approach (including only a single harmonic) yields qualitatively different spectra from the full microscopic fRG+STM results, also ruling out the possibility to distinguish gapped and nodal SC order parameters on the basis of the out-of-plane STM signal alone. Combined fRG and STM method for graphene and cobaltates A graphene monolayer and water-intercalated cobaltates are considered as prototypical examples where, as shown in Fig. 1 , the fRG method predicts the possibility of a chiral d+id SC state. In this manuscript, we propose the combined fRG+STM method as a powerful tool to distinguish between d+id and f-wave order parameters in these materials. 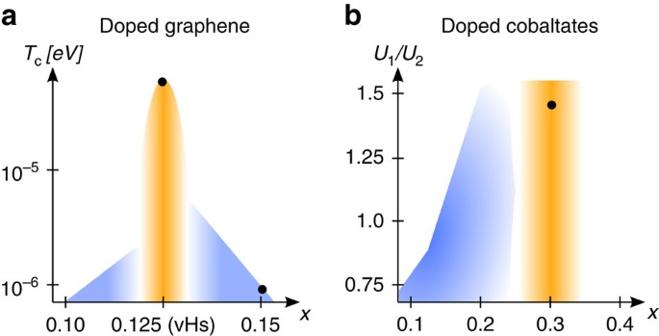Figure 1: Schematic phase diagrams obtained from fRG calculations. The phase diagram for doped graphene (a) and for water-intercalated sodium cobaltates (b). The competing phases consist of the chiral superconducting d+id phase in the singlet channel, the f-wave phase in the triplet channel as well as the competition with a spin-density wave (SDW) phase. In the orange area the d+id superconducting phase and the SDW compete (d+id wins near van Hove singularity in graphene or close to perfect FS nesting in cobaltates), whereas in the blue area the two superconducting phases compete. The black dots denote the phase-diagram points for which the TRS-breaking d+id-phase and the TRS-conserving f-phase are calculated and taken as inputs in the STM scheme. For the cobaltates, the doping has been confined for both d+id and f-phases to the valuex≅0.3, where SC has been observed experimentally. Figure 1: Schematic phase diagrams obtained from fRG calculations. The phase diagram for doped graphene ( a ) and for water-intercalated sodium cobaltates ( b ). The competing phases consist of the chiral superconducting d+id phase in the singlet channel, the f-wave phase in the triplet channel as well as the competition with a spin-density wave (SDW) phase. In the orange area the d+id superconducting phase and the SDW compete (d+id wins near van Hove singularity in graphene or close to perfect FS nesting in cobaltates), whereas in the blue area the two superconducting phases compete. The black dots denote the phase-diagram points for which the TRS-breaking d+id-phase and the TRS-conserving f-phase are calculated and taken as inputs in the STM scheme. For the cobaltates, the doping has been confined for both d+id and f-phases to the value x ≅ 0.3, where SC has been observed experimentally. Full size image Starting with the Hamiltonian for the cobaltates (see Methods) which only includes on-site electron–electron interactions, the fRG flow will generate longer-range electron–electron interactions. Since the longer-range electron–electron interactions cause higher-order harmonics to be induced in the d+id-wave SC channel, the in-plane STM signal will show qualitatively new features in comparison with the phenomenological d+id SC channel. This immediately shows the necessity to apply the fRG+STM method. Furthermore, the fRG+STM approach gives a new methodology, which allows for a reliable distinction between the topological d+id and the f-wave SC phase. To fully appreciate the strength of the fRG+STM approach, we first explain the advantages of the fRG method and how the fRG input is fed into the material-oriented STM calculations. In the cobaltates, the fRG starts from a three-orbital model (see Methods), where a core ingredient is the effect of longer-range hoppings, shifting the filling of perfect nesting away from the van Hove filling. The C 6v acts as the decisive symmetry which can yield a chiral d-wave below the critical temperature T C to maximize the condensation energy. Several common features as compared to the cobaltate case can be identified in graphene, such as the role of longer-range hoppings in providing a distinction between van Hove filling and the filling of perfect nesting. In particular, we discuss the chiral d-wave state, which competes with f-wave SC further away from van Hove filling and turns into a SDW state near van Hove filling beyond a certain interaction strength. Of all theoretical approaches, mainly the fRG has been capable of fully describing such a scenario [34] , [35] . More precisely, in graphene, we illustrate the fRG+STM analysis of shorter- and longer-range Hubbard interactions on a generalized honeycomb tight-binding model up to third-nearest neighbour hybridization (see Methods). As seen in Fig. 1a , at the vHS (orange area), chiral d+id pairing competes with, but wins over the SDW channel (details for the underlying band structure and the Hamiltonian are summarized in the Methods). Away from the vHS (blue area), the critical instability scale Λ C , Λ C ∼ T C drops and whether the d+id or the competing f-wave instability is preferred depends on the range of electron–electron interactions. We show differential conductance plots for graphene with short-range Coulomb interactions in this article and long-range Coulomb interactions in Supplementary Fig. 1 and Supplementary Note 1 , because the carrier density and the corresponding range of electron–electron interactions is different due to charge screening for the two different doping situations. At Λ C , which denotes the critical fRG flow parameter, where the leading instability starts to diverge, the different channels such as the SC d+id and f-wave channels are decomposed into different eigenmode contributions and the corresponding gap form factors are obtained (see Methods). They are then used as a microscopic input into the STM procedure. The black dots in Fig. 1 denote the phase-diagram points for which the TRS-breaking d+id-phase and the TRS-conserving f-phase are calculated and taken as inputs in the STM scheme. For the cobaltates ( Fig. 1b ), the doping has been confined for both d+id and f-phases to the value x ≅ 0.3, where SC has been observed experimentally. In the second step the differential conductance of these quasi two-dimensional SC is calculated using a normal metal–insulator–SC (N–I–SC) set-up with the pairing potentials from the fRG calculation. Such a N–I–SC junction, formulated for a δ -function barrier model [46] , is known to imitate very well an experimental STM set-up. This is documented by a variety of applications, where the pairing potentials have been used as a phenomenological ansatz for distinguishing different SC symmetry channels [21] , [46] , [47] , [48] , [49] . The effective barrier-height is represented by , where m , k FN and H denote the electron mass, the Fermi momentum on the normal side, and the barrier potential, respectively. Both in-plane and out-of-plane set-ups are considered, where in the first (second) case the STM lies in (is oriented perpendicular to) the SC plane. Solving, as in previous phenomenological studies, the Bogoliubov–de Gennes equations with the appropriate boundary conditions, but now with the momentum dependent microscopic pairing potentials, the coefficients (probabilities) for Andreev reflection r A and normal reflection r N are obtained. Via the Blonder–Tinkham–Klapwijk (BTK)-formula [50] , the conductance is given by: for the quasiparticle injection with energy E =−e V , where V is the bias voltage, and θ is the incident angle with respect to the interface ( Fig. 2 ). More details for the calculation of the normalized differential conductance can be found in the methods. Here it suffices to note that the conductance contains two distinct pairing potentials Δ + and Δ − . They correspond to the effective pairing potentials for transmitted electron-like quasiparticles (ELQ) and hole-like quasiparticles (HLQ), respectively, as shown in Fig. 2 . The total conductance is given by integrating the angle-resolved conductance of equation (1) over all transverse momenta, which are the independent modes. Except in the low-barrier (small Z 0 −) limit, which is not of interest here (our choice of Z 0 =5 corresponds to a high barrier), the conductance peak corresponds to the Andreev bound-state energy level, which is formed at the edge of the SC (see Fig. 3 of ref. 46 ). 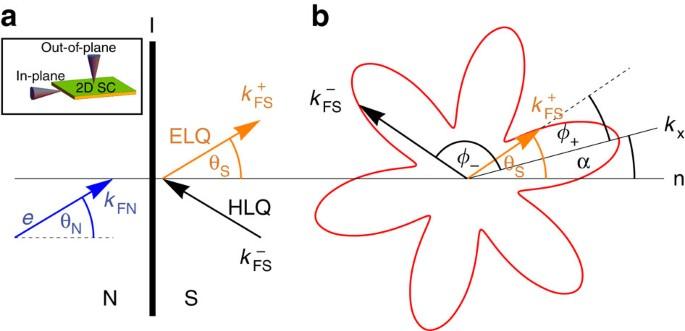Figure 2: Geometry of the STM set-up. (a) Angle definitions for the normal metal (N)—insulator (I)—superconductor (SC) junction. An incident electron on the normal side is characterized by the angleθN(with respect to the surface normal n). On the superconducting side, transmitted electron-like quasiparticles (ELQ) have the momentum vector(angleθSwith respect to the surface normal n) and hole-like quasiparticles (HLQ) have. The inset shows the set-up: The STM tip can be placed either in-plane or out-of-plane with respect to the quasi two-dimensional (2D) SC. (b) Angle definitions for the pair potential. The angleφ+(φ−) for ELQ (HLQ) is measured with respect to thekxdirection of the pair potential, that can be tilted by an angle α with respect to the surface normal n. Note, that ELQ and HLQ experience different effective pair potentials. Figure 2: Geometry of the STM set-up. ( a ) Angle definitions for the normal metal (N)—insulator (I)—superconductor (SC) junction. An incident electron on the normal side is characterized by the angle θ N (with respect to the surface normal n). On the superconducting side, transmitted electron-like quasiparticles (ELQ) have the momentum vector (angle θ S with respect to the surface normal n) and hole-like quasiparticles (HLQ) have . The inset shows the set-up: The STM tip can be placed either in-plane or out-of-plane with respect to the quasi two-dimensional (2D) SC. ( b ) Angle definitions for the pair potential. The angle φ + ( φ − ) for ELQ (HLQ) is measured with respect to the k x direction of the pair potential, that can be tilted by an angle α with respect to the surface normal n. Note, that ELQ and HLQ experience different effective pair potentials. 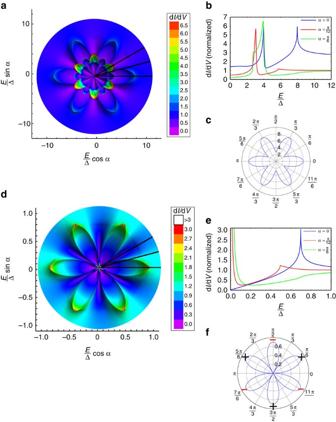Figure 3: Differential conductance spectra (dI/dV) and corresponding pairing potentials for graphene. Panels (a), (b) and (d), (e) show the differential conductance spectra for the d+id pairing phase and the f pairing phase, respectively. The corresponding pairing potentials are shown in panels (c) and (f) as a polar plot of the absolute value of the pairing potential. The differential conductance spectra, obtained in the in-plane set-up simulating an STM experiment (panels (a) and (d)), are plotted as a function of the quasiparticle energyE(radial axis, normalized by the reference bandgap Δ) and the angleαbetween the interface normal and thekx-direction of the pairing potential (polar axis). The differential conductance is normalized by the conductance of a N–I–N junction in the same geometry. Differences in brightness of the colours are due to the plot style. The black lines indicate angles α, for which the cross-sections are shown in panels (b) and (e). The cut forα= 0 in (b) was scaled by a factor of 50. Full size image Figure 3: Differential conductance spectra ( dI / dV ) and corresponding pairing potentials for graphene. Panels ( a ), ( b ) and ( d ), ( e ) show the differential conductance spectra for the d+id pairing phase and the f pairing phase, respectively. The corresponding pairing potentials are shown in panels ( c ) and ( f ) as a polar plot of the absolute value of the pairing potential. The differential conductance spectra, obtained in the in-plane set-up simulating an STM experiment (panels ( a ) and ( d )), are plotted as a function of the quasiparticle energy E (radial axis, normalized by the reference bandgap Δ) and the angle α between the interface normal and the k x -direction of the pairing potential (polar axis). The differential conductance is normalized by the conductance of a N–I–N junction in the same geometry. Differences in brightness of the colours are due to the plot style. The black lines indicate angles α, for which the cross-sections are shown in panels ( b ) and ( e ). The cut for α = 0 in ( b ) was scaled by a factor of 50. Full size image Differential conductance spectra for the in-plane set-up In the previous sections a theory for the tunnelling spectroscopy of a N–I–SC junction, combined with the microscopic fRG derivation of the underlying pairing potentials, was proposed as a new and efficient tool for identifying, in particular, a chiral SC state with broken TRS. The differential conductance for the in-plane set-up is shown in polar plots ( Figs 3a,d and 4a,d ), where the radial axis is the quasiparticle excitation energy normalized by the superconducting energy (gap) scale Δ, which is a common energy scale obtained from fRG. α denotes the angle between the interface normal (n) and the k x direction ( Fig. 2 ). The absolute value of the pairing potential is also shown in a polar plot to compare it with the differential conductance. For each phase, cross-sections at three different angles α are given ( Figs 3b,e and 4b,e ). The chosen angles are indicated by black lines in the d I /d V characteristics. 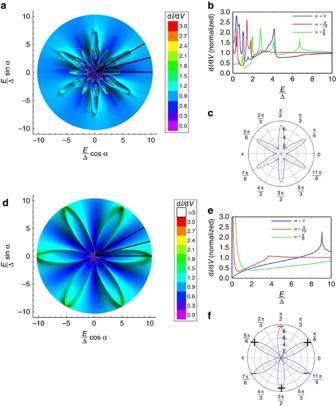Figure 4: Differential conductance spectra (dI/dV) and corresponding pairing potentials for the cobaltates. Panels (a), (b) and (d), (e) show the differential conductance spectra for the d+id pairing phase and the f pairing phase. The corresponding pairing potentials are shown in panels (c) and (f) as a polar plot of the absolute value of the pairing potential. The differential conductance spectra, obtained in the in-plane set-up simulating an STM experiment (panels (a) and (d)), are plotted as a function of the quasiparticle energyE(radial axis, normalized by the reference bandgap Δ) and the angle α between the interface normal and thekx-direction of the pairing potential (polar axis). The differential conductance is normalized by the conductance of a N–I–N junction in the same geometry. Differences in brightness of the colours are due to the plot style. The black lines indicate anglesα, for which the cross-sections are shown in panels (b) and (e). Figure 4: Differential conductance spectra ( dI / dV ) and corresponding pairing potentials for the cobaltates. Panels ( a ), ( b ) and ( d ), ( e ) show the differential conductance spectra for the d+id pairing phase and the f pairing phase. The corresponding pairing potentials are shown in panels ( c ) and ( f ) as a polar plot of the absolute value of the pairing potential. The differential conductance spectra, obtained in the in-plane set-up simulating an STM experiment (panels ( a ) and ( d )), are plotted as a function of the quasiparticle energy E (radial axis, normalized by the reference bandgap Δ) and the angle α between the interface normal and the k x -direction of the pairing potential (polar axis). The differential conductance is normalized by the conductance of a N–I–N junction in the same geometry. Differences in brightness of the colours are due to the plot style. The black lines indicate angles α , for which the cross-sections are shown in panels ( b ) and ( e ). Full size image More specifically, the differential conductance spectra, obtained in the in-plane set-up simulating an STM experiment, are presented for the d+id- and f-pairing phases of graphene ( Fig. 3 ) and for water-intercalated sodium cobaltates ( Fig. 4 ). Comparing the conductance spectra (d I /d V ) for the d+id-pairing phase ( Fig. 3a ) with the f-pairing phase ( Fig. 3d ), it becomes clear why the fRG+STM calculation is an ideal tool to distinguish a d+id-wave TRS-broken phase from a f-wave TRS-conserving phase. In graphene, for the chiral d+id case, the polar d I /d V intensity plot displays, in addition to the outer structure (which maps the local density of states with the peaks appearing at the local pairing potentials—compare with the pairing potential in Fig. 3c ) an inner structure for energies smaller than the superconducting bandgap, which is called sunflower structure in what follows. It is this inner coloured sunflower structure which immediately signals the presence of a TRS-broken SC state. A similar, but even more complicated inner structure for the cobaltates (below the bandgap E =6.7Δ) is again the sign of broken TRS ( Fig. 4a ). To understand the physical content of these differential conductance spectra for the d+id and f-pairing phases in more detail, let us summarize what kind of physical quantity the tunnelling spectroscopy is detecting. The energy level giving the conductance peak is determined by a quantum condition of the bound quasiparticles (QPs) in a pseudo-quantum well. This quantum well is formed by the N–I–SC junction ( Fig. 2a ), where an electron injected from the N-side is transmitted into the SC ejecting an Andreev HLQ. This hole-like quasi-particle with its wave vector scatters into an ELQ with after reflection from the I–SC interface, with a corresponding change in the effective pair potentials from to at the insulator (ref. 46 , in particular Fig. 3 therein). The bound states form at the interface and the tunnelling electrons in the N–I–SC junction flow via these bound states. These states have been shown in earlier work by Tanaka et al. [51] to converge to the edge states of the SC (trivial or non-trivial) in the large barrier-height limit (which is considered here). We use the bulk order parameters for the matching. However, since we introduce an interface, the topological edge states for the d+id pairing phase appear naturally due to the bulk-edge correspondance (ref. 49 ). The analogy with the QP and their Andreev reflection in a pseudo-quantum well is useful for a transparent physical understanding of the inner sunflower structure appearing in the STM spectra of Figs 3a and 4a , as discussed below. The quantum-well analogy has been suggested by Kashiwaya et al. [46] and shows the equivalence of the bound QP condition of the N–I–SC junction with that of QPs in a SC–N–SC structure (with thickness of N → 0 and no difference of the superconducting phase across the junction), in which the pair potentials of the two superconductors are Δ + and Δ − , respectively. The QPs in the pseudo-quantum well (normal region N) are confined if their energies are less than the amplitudes of both pair potentials, this is E <min(|Δ + |,|Δ − |). In the SC–N–SC junction, the bound QPs travel along a closed path by repeating Andreev reflections at both N–SC and SC–N interfaces. This is, then, equivalent to the formation of the Andreev bound states in the N–I–SC junction, as explained in the paragraph above and in refs 46 , 49 . The corresponding peak condition for the bound QPs, which was first reported by Kashiwaya et al [46] , is given in equation (7) of the methods. Here we consider its general properties, which help to understand the occurrence of the outer peaks and that of the inner sunflower structure in Figs 3a,d and 4a,d . For Δ − = Δ + , the peak condition, given in equation (7), is fulfilled if the energy E of the injected particle is E =|Δ ± |. Consequently, a peak at the bandgap occurs, which is the outer structure in Figs 3a,d and 4a,d . We call this peak the local bandgap peak, since as shown in these figures, the bandgap value depends on the (local) polar angle ϕ . The polar angle is defined as , with k x ( φ )= k F ( φ ) cos φ and k y ( φ )= k F ( φ ) sin φ and is given for ELQ by φ + = θ S − α and for HLQ by φ − = π − θ S − α ( Fig. 2 ). α denotes the angle between the interface normal (n) and the k x -direction and θ S is the angle between the interface normal and the momentum of the ELQ in the SC. The zero-energy Andreev bound state (ZEBS) with E =0 occurs if the phase difference of the pair potentials Δ + and Δ − , denoted by Φ + −Φ − (where Δ ± =|Δ ± |exp( i Φ ± )), in equation (7) is ± π . Φ ± simplifies to Φ ± = φ ± , if k F does not depend on φ and a d+id pair potential with equal mixing of and d xy on the square lattice is considered. The novel aspect of more harmonics and an angle dependent k F leads to a more complicated peak structure in the differential conductance curves (see Figs 3 and 4 and Supplementary Fig. 1 ). One possibility to fulfil Φ + −Φ − =± π is Δ + =−Δ − for purely real pair potentials. The resulting ZEBS are seen in our fRG+STM calculations for the f-pairing phase in Fig. 3d , as well as in Fig. 4d . However, for a complex d+id pairing potential, the condition Δ + =−Δ − is not sufficient. This is exactly the situation encountered for the inner sunflower structure of the d+id order parameter shown in Fig. 3a : Since and , the phase difference between the two pair potentials is not restricted to multiples of π . Thus, the peak position moves between 0 and min(|Δ + |,|Δ − |), depending on the relation of Δ + , Δ − and the angle α . This peak is also called double-split peak, since the zero energy conduction peak is split into two peaks positioned symmetrically at positive and negative finite energies. This confirms the usefulness of the analogy with the pseudo quantum well and implies that indeed the QP in the quantum well are only confined if their energies are less than the amplitudes of both pair potentials. Our differential conductance for the full (fRG+STM) calculations of the d+id order parameter on the honeycomb lattice is very different from what is usually done in a phenomenological STM approach. There, one considers only the first harmonic in the superconducting gap, in other words one assumes only short-range (nearest-neighbour) electron—electron interactions entering the pairing (gap) function. The ‘phenomenological’, nearest-neighbour, d I /d V plot is shown in Supplementary Fig. 2 for the in-plane set-up ( Supplementary Note 2 ) and is even qualitatively different from the one obtained in Fig. 4a of this manuscript for the realistic d I /d V signal, here for cobaltates. The difference between realistic material-oriented and phenomenological approaches comes from the fact that although the high-energy Hamiltonian (for the cobaltates, equation (3) of the Methods) includes only on-site electron–electron interactions, the fRG flow will induce longer-range electron–electron pairings beyond nearest-neighbours in the pairing channel. Therefore, the full (fRG+STM) calculations include additionally also these higher-order interactions (higher harmonics). They give rise to a quite complex ‘sunflower’ structure of the d+id order parameter. Therefore, the fRG procedure provides qualitatively new insight into the differential conductance and is obviously essential if one wants to uniquely resolve a topological SC state. In contrast to the conductance curves of the d+id pairing phases, that reveal clear signatures of broken TRS, the conductance curves of the f pairing phases contain zero energy peaks, which are present due to conserved TRS. These zero energy peaks are seen in the cuts ( Figs 3e and 4e , Supplementary Fig. 1e for a zoom for small quasiparticle energies, displaying the ZEBS in white). As discussed already above, these peaks originate from an antisymmetric pairing Δ + =−Δ − . Further, the differential conductance is rotated with respect to the order parameter. The physical reason for this effect is a lack of inversion symmetry for the f order parameter with respect to the origin of the k x – k y plane (let us mention that this inversion is preserved for both real and imaginary parts of the d+id order parameter). This lack of inversion symmetry and the corresponding rotation of the f order parameter can be easily understood, considering for example graphene ( Fig. 3d ) at an angle . Then, ELQ exhibit a pair potential of and HLQ of . Using the pair potential (the signs of the pair potentials for a phase difference of π are opposite in Fig. 3f ), we find Δ + =−Δ − , giving rise to a zero energy peak, which is indeed found in the conductance spectrum at . Let us add a few more details, concerning the results in Figs 3 and 4 . Figure 3 shows the differential conductance spectra and the pairing potentials for d+id and f pairing phases of graphene with short-range Coulomb interactions at the vHS where the screening is very effective. Corresponding d I /d V characteristics for a larger doping x =0.15 (long–range Coulomb interactions) are presented in Supplementary Fig. 1 (see also Supplementary Note 1 ). A given α direction corresponds to a specific surface, which can be expressed with Miller indices. Cross-sections for α =0 and correspond to Miller indices (1,−1,0) and (1,0,0) for cobaltates and, respectively, (1,−1) and (1,0) for graphene. The cross-sections of d I /d V characteristics in Figs 3e and 4e show that the width of the zero energy peaks is maximal in the maximum bandgap directions of the pairing potential (given by , ), in which the condition of antisymmetric pairing is fulfilled for all incident angles θ (angle between the incident momentum and the interface normal, see Methods). In general, the height of the peaks depends on how many incident angles θ contribute to the resonance for a given α direction. In the case of the cobaltates, the gap is very anisotropic and more harmonics contribute than for graphene. Consequently, the number of incident angles contributing to a resonance is smaller, giving a smaller peak height. Summarizing, the in-plane set-up is sensitive to the magnitude and the phase of the pair potential, and allows to distinguish the different pairing phases (d+id and f). While the f-wave pairing phase gives zero energy peaks typical for order parameters with conserved TRS, the signature of broken TRS can be clearly seen in the sunflower structure in the differential conductance spectrum of the d+id paring phase of our prototypical examples. 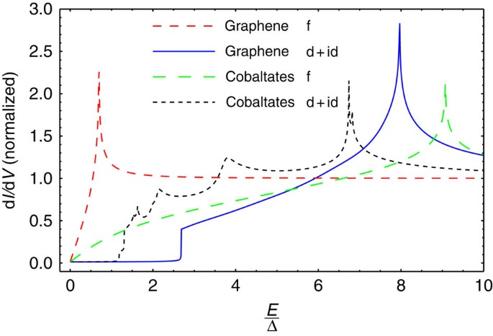Figure 5: Differential conductance (dI/dV) for the out-of-plane set-up at zero temperature. The differential conductance is normalized by the conductance of a N–I–N junction in the same geometry and shown as a function of the quasiparticle energyEnormalized by the reference bandgap Δ. The curves of the d+id and f pairing phases are given for graphene and the cobaltates. Differential conductance spectra for the out-of-plane set-up Figure 5 shows the differential conductance obtained in the out-of-plane set-up for the d+id and f pairing phases of graphene and the cobaltates. The out-of-plane set-up shows only the density of states features since the information about the phase and the in-plane angle dependence of the pairing potential is integrated out. The density of states induces peaks at energies that match the maximum pairing potential, causing maximal Andreev reflection and a peak in the d I /d V characteristics. For the d+id pairing phase of graphene there is only one peak at the maximum pairing potential (8Δ). On the other hand, the differential conductance curve of the d+id pairing phase of the cobaltates displays a number of peaks, each one corresponding to a local maximum (or saddle point) of the pairing potential. This signature is again a manifestation of the strongly anisotropic d+id pairing phase of the cobaltates. Figure 5: Differential conductance ( dI / dV ) for the out-of-plane set-up at zero temperature. The differential conductance is normalized by the conductance of a N–I–N junction in the same geometry and shown as a function of the quasiparticle energy E normalized by the reference bandgap Δ. The curves of the d+id and f pairing phases are given for graphene and the cobaltates. Full size image Since the f pairing potentials are nodeless in some specific directions, the d I /d V curves for the f-phases grow with the excitation energy until the peak for the maximal pairing potential is reached. For the d+id pairing phase, a kink is observed at the minimum pairing potential value, because Andreev reflection occurs for some directions in momentum space. Furthermore, for the d+id pairing phases, there is no conductance observed below the minimum pairing potential value, because normal electron reflection is the only process in this regime. This region of zero conductance, in many cases, is a signature of a gapped phase, that allows to distinguish between gapless and gapped pairing potentials. In our role-model system cobaltates ( T C =5 K [39] ), however, as shown in Supplementary Fig. 3a,b (differential conductance curves as a function of temperature for the out–of-plane STM configuration) this is not the case for temperatures of the order of a few Kelvins (0.25Δ≤ k B T < k B T C ). This originates from the fact that the out–of-plane set-up is only sensitive to the density of states, and the temperature broadening is of the order of the small d+id SC gap. In contrast, in the in-plane STM set-up ( Supplementary Fig. 3c,d and Supplementary Note 3 ), the Andreev bound states in the d+id order parameter are robust against temperature smearing. That is exactly the reason why one needs not only the out-of-plane but also the in-plane STM set-ups to identify topological superconductivity in realistic materials. Our results show that the combination of the fRG pairing input with the STM spectroscopy analysis allows for an unambiguous characterization of the SC state and its pairing symmetry, starting from a microscopic, in principle a priori description of the interacting Hamiltonian. The relevance of this combination becomes especially clear when considering the possibility of unconventional SC on hexagonal lattices. In many layered compounds, which are candidates for electronically driven (high T C ) SC, the atoms form a square lattice. For the intensively studied square-lattice material classes, such as the cuprates and pnictides, experimental evidences and theoretical descriptions have already provided a rich picture. A celebrated example is, of course, the d-wave symmetry of the SC state in the cuprates, by which its momentum profile of the SC gap points directly to the decisive role of electronic correlations for the pairing mechanism. The situation is rather different for unconventional SC in hexagonal systems. In only a few hexagonal materials, the origin of SC can so far be assigned unambiguously to electronic interactions, partly due to the often occurring lattice distortions, which make a phonon-driven scenario of SC more likely. (It can even be such that electronic correlations strengthen phonon-induced pairing [52] .) However, there are also compounds, where strong correlations, in combination with a hexagonal lattice symmetry are very likely to induce unconventional SC [53] . Bechgaard salts are certainly candidates for organic unconventional superconductors [54] , [55] . As mentioned before, the pnictide compound SrPtAs has recently attracted substantial attention: it is a multi-layer compound, where Pt and As atoms are arranged in honeycomb rings. Preliminary evidence for a TRS-broken SC phase stems from μ-SR data [37] , [42] . Another relevant material class on the triangular lattice are the water-intercalated sodium cobaltates [39] , which are discussed in detail here as one example for the strength of the fRG+STM method. Another promising avenue towards hexagonal Fermi surface (FS) instability may be related to the emerging possibility of creating hexagonal optical lattices with fermionic isotopes [56] , [57] of ultra-cold atomic gases, provided that the limit T < T C , T / T F <<1, where T F is the Fermi temperature, can eventually be reached. The cobaltates, very much like our other example graphene, for which the FS instability study is transferred from the triangular lattice of the cobaltates to the honeycomb lattice, constitute typical examples, where the fRG provides us with an approach to obtain the unbiased phase diagrams of the FS instabilities in all parquet channels. The combination with the STM then elevates the microscopic theory, the fRG, to a new level directly accessible in scanning tunnelling microscopy experiments. This brings us finally to the discussion how to distinguish experimentally between different pairing phases using scanning tunnelling microscopy. While one expects a gap in the d I /d V characteristics for the d+id phase (zero differential conductance until the minimal pairing potential is reached), the differential conductance increases continuously with energy from zero for the gapless f-pairing phase. However, the resolution in an STM experiment is mainly limited by the temperature. For realistic temperatures of 3–4 K< T C (for cobaltates), the resolution is typically around 0.25–0.3 meV. If the superconducting energy scale Δ is of the order of 1 meV, as expected from a rough estimate within fRG, it might be already very difficult to distinguish between d+id and f wave pairing phases for cobaltates in the out-of-plane STM set-up (see Supplementary Fig. 3a,b ). However, for the small gap of the highly anisotropic d+id pairing potential, a careful analysis of, additionally, the in-plane STM set-up should help resolving all ambiguities. Here for both the cobaltates and graphene, one can clearly see the zero-energy peaks for the TRS-preserving SC state, in contrast to the d+id pairing phase where the characteristic inner sunflower structure is a fingerprint of the chiral SC state. Details of the fRG calculations The strength of the fRG technique is evidenced in both graphene and cobaltate examples: both display near-nested Fermi surfaces [34] , [36] , where SC has to compete with SDW and charge-density wave instabilities. The emergent orders are then determined in an unbiased manner by the renormalization group flow of the corresponding susceptibilities and of the related interaction channels to low energies at the instability level, which is ∼ k B T C in the SC channel [28] . The high-energy starting point is given by the Hamiltonian which is accurately determined for the band structure part H 0 (typically taken from a fit to an a priori density functional theory calculation) and for the interaction H int (taken for example from a constrained random phase approximation). Details of the parameter choices can be found in ref. 28 . For the cobaltates, the Hamiltonian includes three hybridized orbitals per site (d xy , d yz , d zx ) and reads [58] where denotes the electron creation operator with spin σ =↑, ↓ and orbital α at site i. The occupation number is defined as . In addition, t represents the hopping mediated by O pz orbitals and corresponds to a direct Co-Co-hopping, D is the crystal-field splitting, and μ the chemical potential. These parameters are set to t =0.1 eV, and D =0.10 eV. The parameters U 1 =0.37 eV and U 2 =0.25 eV are intraorbital and interorbital Coulomb interactions, respectively. The remaining interaction parameters are J H = J p =0.07 eV for Hund’s rule coupling J H and pair hopping J p . In graphene, the tight-binding Hamiltonian H 0 is where . is the creation operator for an electron with spin σ at site i , μ denotes the chemical potential, and t 1 ⋯ 3 is the hopping strength for nearest neighbour (1), second nearest neighbour (2) and third nearest neighbour (3) hopping. Coulomb interaction is included by a long-range Hubbard-type Hamiltonian H int with where U 0 ⋯ 2 gives the Coulomb repulsion scale from on-site (0) to second nearest neighbour (2) interactions, respectively. The near-degeneracy between SC and density-wave orders is strongly influenced by a subtle interplay between deviations from perfect nesting (taken into account in H 0 of equations (3) and (4) via longer-ranged hopping terms) and the absolute interaction scale. Similarly, the near-degeneracy between TRS-breaking d+id SC order and TRS-preserving f-wave SC order is affected both by the Fermi surface topology and by the interaction terms. For example, in graphene at the vHS, we assume perfect screening and consider a Hubbard-type of Hamiltonian with on-site interaction U 0 =10 eV. Here a d+id SC phase is found ( Fig. 1a ). Away from the vHS ( x =0.125), we take longer-ranged Coulomb interactions into account ( U 1 / U 0 =0.45, U 2 / U 0 =0.15). The latter interactions determine, in particular, whether the competing f-wave SC instability is preferred. Using the above Hamiltonian (equation (2)), we then employ the fRG and study how the renormalised interaction evolves under integrating out high-energy fermionic modes. At weak to moderate electron–electron interactions, this flow is accurately described by the fRG method, where one considers the flow of a function f (instead of a parameter) such as the interaction vertex, depending on four momenta [28] . The renormalised interaction vertex (the 4-point function) is V Λ ( k 1 , k 2 , k 3 , k 4 ), where the flow parameter Λ corresponds to the effective or low-energy scale temperature and k i label the incoming and outgoing momenta and the associated band indices. The starting conditions of the renormalization group are given by the bare interactions as contained in equations (3) and (5), at an energy scale of the order of the bandwidth. Following the flow (we are using the temperature-flow fRG [59] ) of the 4-point function (4PF) V Λ down to low energies, the diverging channels at Λ C then signal the nature of the instability, with Λ C providing an upper bound for T C . At this low-energy scale, the flow has to be stopped and the remaining modes be treated with a different approach. We resort to a mean-field scheme, where the effective interaction determines the SC gap function. This is a standard procedure, which has been used in many applications (for example, ref. 28 ). The phase diagram for graphene is plotted in Fig. 1a . It displays the critical instability scale Λ C ∼ T C as a function of doping. The phase diagram for the water-intercalated sodium cobaltates is presented in Fig. 1b as a function of doping and interaction ratio. We note that, when the nesting of the FS is optimal, singlet d+id SC competes with, but wins over strong SDW fluctuations. On the other hand, in the proximity of ferromagnetic fluctuations (which appear in the cobaltate case in Fig. 1b for large interaction ratios U 1 / U 2 , where the large density of states (DOS) at the vHS promotes fluctuations with zero-momentum transfer), triplet SC with a f-wave gap form factor is dominant. The 4PF V Λ ( k ,− k , q , − q ) in the Cooper channel is, then, decomposed into different eigenmode contributions [28] as where i is a symmetry decomposition index. The leading instability of that channel corresponds to an eigenvalue first diverging under the flow of Λ. is the SC form factor of pairing mode i , which tells us about the SC pairing symmetry and hence gap structure associated with it. In the fRG, from the final Cooper channel 4PFs, this quantity is computed along the discretized FSs. is the gap function which enters the BTK formula (equation (1)) for the conductance (as an example the harmonics for graphene with the short-range electron–electron interactions are shown in Supplementary Methods ). Details of the STM calculations For the STM-part of the calculation, we use the N–I–SC junction set-up and solve the Bogoliubov–de Gennes equations for the normal and the superconducting parts. The insulator is modelled by a delta-Dirac potential barrier with strength H (ref. 46 ). We apply the approximation, that the quasiparticle excitation energy E and the maximum absolute value of the pairing potential max{|Δ|} are much smaller than the Fermi energy E F . Consequently, the pairing is only relevant close to the Fermi surface. Within these approximations, the wave function obtained by solving the Bogoliubov–de Gennes equations ( Supplementary Methods ) is independent of the dispersion relation of the material (we assume to have a quadratic term in the dispersion). We use the continuity of the wave function at the interface and the matching of the derivative of the wave functions of the normal and the superconducting side to obtain the coefficients for Andreev ( r A ) and normal ( r N ) reflection. The total conductance of the N–I–SC junction is obtained by integrating the BTK conductance over all independent contributions, which is integrating over all k y in our in-plane set-up. We normalize the conductance by the conductance of a N–I–N junction in the same geometrical set-up. A peak in the conductance spectrum is obtained, if the following condition, first reported by Kashiwaya et al. [46] is fulfilled where , Φ ± =arg(Δ ± ) and E denotes the quasiparticle excitation energy. In general, Φ ± ≠ φ ± because k F depends on φ . However, for the generic d+id pair potential, Φ ± = φ ± . How to cite this article: Elster, L. et al. Accessing topological superconductivity via a combined STM and renormalization group analysis. Nat. Commun. 6:8232 doi: 10.1038/ncomms9232 (2015).